The landscape of somatic mutations in epigenetic regulators across 1,000 paediatric cancer genomes Studies of paediatric cancers have shown a high frequency of mutation across epigenetic regulators. Here we sequence 633 genes, encoding the majority of known epigenetic regulatory proteins, in over 1,000 paediatric tumours to define the landscape of somatic mutations in epigenetic regulators in paediatric cancer. Our results demonstrate a marked variation in the frequency of gene mutations across 21 different paediatric cancer subtypes, with the highest frequency of mutations detected in high-grade gliomas, T-lineage acute lymphoblastic leukaemia and medulloblastoma, and a paucity of mutations in low-grade glioma and retinoblastoma. The most frequently mutated genes are H3F3A , PHF6 , ATRX , KDM6A , SMARCA4 , ASXL2 , CREBBP , EZH2 , MLL2 , USP7 , ASXL1 , NSD2 , SETD2 , SMC1A and ZMYM3 . We identify novel loss-of-function mutations in the ubiquitin-specific processing protease 7 (USP7) in paediatric leukaemia, which result in decreased deubiquitination activity. Collectively, our results help to define the landscape of mutations in epigenetic regulatory genes in paediatric cancer and yield a valuable new database for investigating the role of epigenetic dysregulations in cancer. Genome-wide mutation profiling of paediatric cancer has yielded important insights into the molecular pathology of the major subtypes of cancer seen in children [1] . Two general observations to emerge from these studies are that paediatric cancers on average contain fewer somatic mutations than comparable tumours occurring in adults; and that genes that encode proteins involved in epigenetic regulation are mutated at a high frequency in a subset of paediatric cancers. A striking example of the latter are mutations in histone 3 ( H3F3A , encoding H3.3 and HIST1H3B , encoding H3.1) that cause a p.Lys27Met amino-acid substitution in up to 78% of diffuse intrinsic pontine glioma—a highly aggressive subtype of paediatric brain tumour [2] , [3] . Additional epigenetic regulators recurrently mutated in paediatric cancers include CREBBP , EED , EP300 , EZH2 , PHF6 and SETD2 in acute lymphoblastic leukemia [4] , [5] , [6] ; CHD7 , HDAC9 , KDM4C , KDM6A , MLL2 , SMARCA4 and ZMYM3 in medulloblastoma (MB) [7] ; and ATRX in neuroblastoma and high-grade glioma (HGG) [2] , [8] . To extend these observations, we determine the frequency of somatic mutations in genes directly implicated in epigenetic regulation across each of the major subtypes of paediatric cancer as part of the St Jude Children’s Research Hospital–Washington University Pediatric Cancer Genome Project [1] . A total of 633 epigenetic regulatory genes in 1,020 paediatric cancers representing 21 different cancer subtypes including brain tumours, solid tumours and leukaemias are sequenced. Our comprehensive analysis helps to define the landscape of mutations in epigenetic regulatory genes in paediatric cancer and provides a database that should be of significant value in elucidating the role of epigenetic dysregulation in cancer. Somatic mutations in epigenetic regulatory genes The 633 epigenetic regulatory genes analysed in this study include enzymes that covalently modify histones including histone writers ( n =159) and histone erasers ( n =55); the proteins that bind histone writers ( n =65) or histone erasers ( n =20); histones ( n =88); histone readers ( n =116); chromatin remodellers ( n =72); and enzymes that covalently modify DNA ( n =58) ( Fig. 1a , Supplementary Data 1 ). 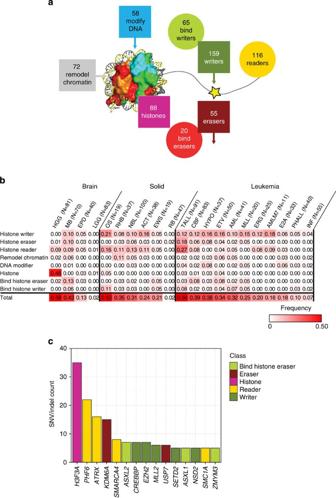Figure 1: The landscape of somatic mutations in epigenetic regulators in 21 paediatric cancer subtypes. (a) Eight classes of epigenetic genes were interrogated across the cohort (histone writer, bind histone writer, histone eraser, bind histone eraser, histone, histone reader, chromatin modifier and DNA modifier), with the numbers of genes within each class indicated. (b) Fraction of tumours in each cancer subtype with at least one mutation in each class of epigenetic genes. Only sequence mutations (that is, SNVs and indels) with a MAF >0.3 (that is, present in the dominant clone) were included in the analysis. Abbreviations are defined in Table 1. (c) Top 15 most frequently mutated genes are colour coded by class. These genes were sequenced in 1,020 paediatric cancers representing 21 different cancer subtypes including brain tumours (4 subtypes), solid tumours (6 subtypes) and leukaemias (11 subtypes; Table 1 ). DNA samples from both tumour and matched germ line were analysed by either whole-genome sequencing (WGS, n =434), whole-exome sequencing (WES, n =244) or custom-designed capture sequencing of all coding exons of the 633 genes (CC, n =426; Table 1 and Supplementary Data 2 ). The average read depth for WGS, WES and CC is 30x, 100x and 342x, respectively. Across the entire cohort, 96.7% of the coding exons of the 633 genes had coverage >20x. Because of the variation in sequencing methods used across the cohort, we limited our mutation analyses to the detection of single-nucleotide variants (SNVs) and small insertions/deletions (indels). This analysis yielded a >90% power to detect mutations that occurred with a mutant allele fraction (MAF) of ≥0.3, and thus focuses on mutations in the dominant malignant clone ( Supplementary Fig. 1 ; Supplementary Data 3 and 4 ). All identified non-silent coding region mutations were experimentally validated by an independent sequencing platform resulting in a total of 668 validated somatic mutations, with 62% (414) occurring with a MAF >30%. Figure 1: The landscape of somatic mutations in epigenetic regulators in 21 paediatric cancer subtypes. ( a ) Eight classes of epigenetic genes were interrogated across the cohort (histone writer, bind histone writer, histone eraser, bind histone eraser, histone, histone reader, chromatin modifier and DNA modifier), with the numbers of genes within each class indicated. ( b ) Fraction of tumours in each cancer subtype with at least one mutation in each class of epigenetic genes. Only sequence mutations (that is, SNVs and indels) with a MAF >0.3 (that is, present in the dominant clone) were included in the analysis. Abbreviations are defined in Table 1. ( c ) Top 15 most frequently mutated genes are colour coded by class. Full size image Table 1 Paediatric tumour data set. Full size table Of the 633 genes, 62 were recurrently mutated across the patient cohort, with an additional 128 genes mutated in a single case ( Supplementary Fig. 2 and Supplementary Data 5 ). The paediatric tumours that had the highest frequency of mutations in epigenetic genes were HGGs, T-lineage acute lymphoblastic leukaemia (TALL) and MB (43–59% of cases in these tumour subtypes had a mutation in an epigenetic gene in the dominant tumour clone, Fig. 1b ). Osteosarcoma also exhibited high rates of mutation in epigenetic regulatory genes; however, the high background mutation rate in these tumours suggest that the majority of the epigenetic regulatory gene mutations in this cancer subtype were passenger rather than driver mutations ( Supplementary Data 5 ). Importantly, several paediatric cancers were notable for almost a complete absence of mutations in epigenetic regulators including low-grade gliomas (LGG), retinoblastoma and infant leukaemia ( Fig. 1b ). However, it is important to remember that the majority of infant leukaemias contain a translocation involving the MLL gene and thus have an alteration in a key epigenetic regulator as part of the leukaemia’s initiating lesions [9] . Most frequently mutated epigenetic regulatory genes The most frequently mutated epigenetic regulatory gene in paediatric cancer (mutated in five or more cases) were H3F3A , PHF6 , ATRX , KDM6A , SMARCA4 , ASXL2 , CREBBP , EZH2 , MLL2 , USP7 , SETD2 , ASXL1 , NSD2 , SMC1A and ZMYM3 ( Fig. 1c ; Supplementary Table 1 and Supplementary Data 5 ). Although each of these genes has been implicated in cancer, USP7 , SMC1A and ASXL2 have only been reported to be mutated in a single paediatric case each, and are rarely mutated in adult cancers ( http://cancer.sanger.ac.uk/cosmic ). Importantly, a majority of the top 15 mutated genes were found to be mutated in multiple different paediatric cancer subtypes. The only exceptions were mutations in ASXL2 , NSD2 , PHF6 , SETD2 and USP7 , which were identified in leukaemias but not in brain or solid tumours. Mutations in at least one of the top 15 genes were found in 23% of the paediatric brain tumours, 15% of paediatric leukaemias, but only in 7% of paediatric solid tumours. When we extend this analysis to all recurrently mutated epigenetic regulators (mutated in two or more cases), brain tumours (30%) and leukaemias (30%) share the highest frequency of cases containing mutations in epigenetic regulators, followed by paediatric solid tumours (17%). Consistent with previous reports, the identified mutations in PHF6 , KDM6A , ATRX , MLL2 , CREBBP , SETD2 , SMARCA4 , ASXL2 , ASXL1 and ZMYM3 are predicted to result in a loss-of-function ( Supplementary Table 1 ). By contrast, the NSD2 p.E1099K mutation has recently been shown to lead to enhanced histone methyltransferase activity [10] , whereas the p.K27M mutation in H3F3A eliminates the ability of this residue to undergo normal regulatory post-translational modifications and confers a gain-of-function activity that leads to a block in the trimethylation of all H3 in the cell including the wild-type protein [11] , [12] . Although both activating and inactivating mutations of EZH2 have been previously reported [6] , [13] , we primarily detected EZH2-inactivating mutations in paediatric cancer. Finally, although the functional significance of the identified cohesion subunit SMC1A missense mutations remains to be determined, some of the identified somatic mutations have been observed as germ line mutations in patients with Cornelia de Lange syndrome [14] . The most frequently mutated epigenetic proteins in paediatric cancer function within a network of eight epigenetic regulatory complexes that include the Set1 (compass/compass-like) [15] , mixed lineage leukaemia (MLL) [16] , activating signal cointegrator-2 containing (ASCOM) [17] , nucleosome remodelling and deacetylation (NuRD) [18] , polycomb repressor 2 (PRC2) [19] , the SWI/SNF containing (BAF/PBAF) [20] , CREBBP/EP300 (CREB) complex [21] and the DNMT1/USP7/UHRF1 (DUU) [22] ( Fig. 2 ; Supplementary Data 5 and 6 ). Nearly half of all proteins contained within these complexes are mutated at least once in paediatric cancer. No significant differences were detected in the frequency of mutations within the BAF/PBAF and inter-related MLL/ASCOM/compass complexes across the paediatric cancer subtypes analysed. By contrast, over half of the mutations within the CREB, PRC2 and NuRD complexes occurred in paediatric leukaemias, and all of the mutations in the DUU complex, which regulates DNA methylation and histone deubiquitination, were identified in leukaemias. Of particular note, novel mutations were observed in the ubiquitin-specific processing protease 7 ( USP7 ). 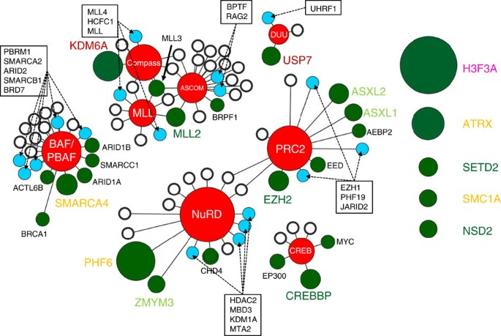Figure 2: Epigenetic complexes affected by recurrently mutated proteins in paediatric cancer. A subset (35%) of the recurrently mutated epigenetic regulatory proteins (green circles) function within one or more of the eight key epigenetic protein complexes (red nodes). Individual somatic mutation were also detected in additional components of these complexes (blue circles), whereas other components were never found to be mutated within our patient cohort (white circles). The size of each green circle is proportional to the number of mutated samples. The distance between the circles and the central complex node indicates whether the protein is a core (short) or transient (long) component of the complex. Recurrently mutated proteins that do not belong to one of these core complexes are presented on the right as unattached circles. The colour of each protein name conforms to the colour scheme for epigenetic regulatory classes presented inFig. 1. Figure 2: Epigenetic complexes affected by recurrently mutated proteins in paediatric cancer. A subset (35%) of the recurrently mutated epigenetic regulatory proteins (green circles) function within one or more of the eight key epigenetic protein complexes (red nodes). Individual somatic mutation were also detected in additional components of these complexes (blue circles), whereas other components were never found to be mutated within our patient cohort (white circles). The size of each green circle is proportional to the number of mutated samples. The distance between the circles and the central complex node indicates whether the protein is a core (short) or transient (long) component of the complex. Recurrently mutated proteins that do not belong to one of these core complexes are presented on the right as unattached circles. The colour of each protein name conforms to the colour scheme for epigenetic regulatory classes presented in Fig. 1 . Full size image Loss-of-function mutations in USP7 The deubiqutinase USP7 has been suggested to lead to the stabilization of several nuclear proteins including the tumour suppressor p53 (ref. 23 ), PTEN [24] , the DNA methyltransferase DNMT1 (ref. 22 ) and histone H2B [25] . Nine USP7 mutations were detected in eight patients in our study ( Fig. 3a ). There were five frameshift mutations (T177fs, V203fs, R340fs, D380fs and D483fs) that would encode truncated proteins that lack the full catalytic domain and four missense mutations (C300R, D305G, A381T, Q821R). Three of the missense mutations occurred within the catalytic domain and based on the crystal structure of USP7, reside at the binding interface between the catalytic domain of USP7 and ubiquitin ( Fig. 3b ), a region that when mutated has been shown to impair ubiquitin binding [26] . C300R is predicted to structurally perturb one side of the USP7 ubiquitin binding pocket, and A381T and D305G alter interactions with key ubiquitin binding residues ( Supplementary Figs 3–5 ). All except one of the USP7 mutations (A381T) were found in TALL resulting in an overall mutation frequency of 8% in TALL. Of the seven TALL cases with a USP7 mutation, none had somatic mutations in TP53 . 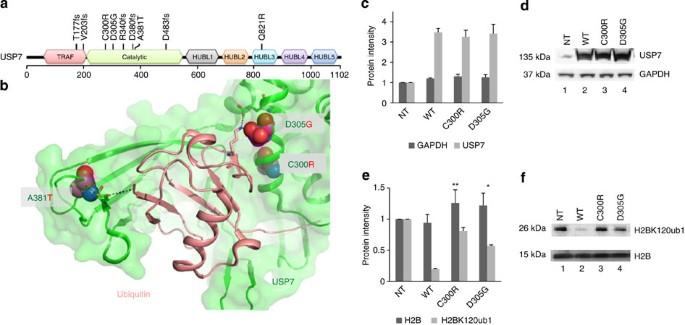Figure 3: Novel ALL-specific mutations of USP7. (a) Location of the identifiedUSP7somatic mutations relative to the TRAF (tumour necrosis factor receptor-associated factor), catalytic and HUBL1-5 (USP7/HAUSP ubiquitin-like domain) domains (coloured red, green, black, orange, teal, purple and blue, respectively). Mutations C300R, D483fs and Q821R occurred at MAF <30%, whereas all other mutations occurred with MAF >30% and thus represent the dominant malignant clone. (b) Location of the missense somatic mutations (C300R, D305G and A381T: magenta space filled) within the USP7 catalytic domain (green cartoon)–ubiquitin (peach cartoon) interface. Specific residues and interactions between USP7 and ubiquitin are shown as sticks and black dots and further described inSupplementary Figs 3–5. (c,d) 293T cells were transfected with USP7 wild-type (WT) or mutant constructs as indicated. Protein extracts were prepared at 72 h post transfection and subjected to western blot analysis using antibodies specific to the indicated proteins. Bars represent mean of protein band intensities of 3 replicates±s.e.m. (e,f). The level of histone H2B ubiquityl Lys120 (H2BK120ub1) and total H2B were detected at 72 h by immunoblot using an antibody specific for mono-ubiquitinated and total H2B. Bars represent mean of protein band intensities of three replicates±s.e.m. NT, untransfected control. The statistical significance of the changes observed between wild type and USP7 mutants were assessed byt-test with *P<0.05 and **P<0.01. Figure 3: Novel ALL-specific mutations of USP7. ( a ) Location of the identified USP7 somatic mutations relative to the TRAF (tumour necrosis factor receptor-associated factor), catalytic and HUBL1-5 (USP7/HAUSP ubiquitin-like domain) domains (coloured red, green, black, orange, teal, purple and blue, respectively). Mutations C300R, D483fs and Q821R occurred at MAF <30%, whereas all other mutations occurred with MAF >30% and thus represent the dominant malignant clone. ( b ) Location of the missense somatic mutations (C300R, D305G and A381T: magenta space filled) within the USP7 catalytic domain (green cartoon)–ubiquitin (peach cartoon) interface. Specific residues and interactions between USP7 and ubiquitin are shown as sticks and black dots and further described in Supplementary Figs 3–5 . ( c , d ) 293T cells were transfected with USP7 wild-type (WT) or mutant constructs as indicated. Protein extracts were prepared at 72 h post transfection and subjected to western blot analysis using antibodies specific to the indicated proteins. Bars represent mean of protein band intensities of 3 replicates±s.e.m. ( e , f ). The level of histone H2B ubiquityl Lys120 (H2BK120ub1) and total H2B were detected at 72 h by immunoblot using an antibody specific for mono-ubiquitinated and total H2B. Bars represent mean of protein band intensities of three replicates±s.e.m. NT, untransfected control. The statistical significance of the changes observed between wild type and USP7 mutants were assessed by t -test with * P <0.05 and ** P <0.01. Full size image To directly assess the functional consequences of the USP7 mutations identified in paediatric ALL, we transfected wild-type and mutant USP7 (C300R and D305G) into 293T cells and assessed their effect on the level of mono-ubiquitinated H2B-K120, a known target of USP7 (ref. 25 ). Transfection resulted in similar levels of expression of the wild-type and mutant USP7 proteins ( Fig. 3c,d and Supplementary Fig. 6 ). As expected, enforced overexpression of wild-type USP7 led to marked reduction in the amount of mono-ubiquitinated H2B-K120 ( Fig. 3e,f and Supplementary Fig. 6 ). By contrast, expression of the USP7 mutants failed to alter the level of mono-ubiquitinated H2B-K120 ( Fig. 3e,f and Supplementary Fig. 6 ). By performing sequence analysis on the entire genomic complement of genes that encode epigenetic regulatory proteins in over 1,000 paediatric cancer samples, we have generated an initial view of the somatic mutational landscape of these genes across 21 different paediatric cancer subtypes, including the predominant forms of leukaemia, brain tumours and solid malignancies seen in the paediatric population. Although our analysis is limited to SNVs and indels, these results demonstrate a marked variation in the frequency of mutations seen in the three major paediatric tumour types, with 30% of paediatric brain tumours and leukaemias containing mutations compared with only 17% of paediatric solid tumours. Moreover, specific subtypes of brain tumours and leukaemias exhibited an exceptionally high frequency of mutations in epigenetic regulator genes including 46% of HGGs with mutations in histone H3 (this frequency increasing to 78% for pontine gliomas); 43% of the MBs and 56% of TALLs with mutations in histone writers, erasers, and readers. At the other end of the spectrum were LGG and retinoblastoma, two tumour types that had almost no mutations within epigenetic regulatory genes. Not only did the frequency of somatic mutation of these genes vary across the tumour types, but also the specific genes mutated showed some variation between tumour types. Focusing on the most commonly mutated genes, which function as part of eight key epigenetic protein complexes including PRC2, NuRD, MLL, ASCOM, compass, BAF/PBAF, CREB and DUU, we observed that over half of the mutations within the CREB, PRC2 and NuRD complexes occurred in paediatric leukaemias, and all of the mutations in the DUU complex were identified in leukaemias. By contrast, no significant differences were detected in the frequency of mutations within the BAF/PBAF and inter-related MLL/ASCOM/compass complexes across the paediatric cancer subtypes analysed. Within the DUU complex, we identified the recurrent somatic mutation of the USP7 gene, which encodes a deubiquitinase that interacts with p53, MDM2, DNMT1/UHRF1 and histones. Although rare, somatic mutations of USP7 have been found in adult cancers ( http://cancer.sanger.ac.uk/cosmic ), our structural modelling predicts that they would be well tolerated and thus likely represent passenger mutations ( Supplementary Fig. 7 and Supplementary Table 2 ). By contrast, in paediatric cancer the majority of USP7 mutations identified are loss-of-function mutations including frameshift mutations within the catalytic domain that would encode truncated USP7 proteins and missense mutations that have reduced deubiquitinase activity. Importantly, the paediatric USP7 mutations were exclusively detected in leukaemias, with six of the seven leukaemias containing a mutation classified as non-ETP (or standard) TALL (6/46 (13%) of non-ETP TALLs contain a mutation in this gene). Defining the key intracellular proteins affected by the altered USP7 function and how these changes specifically contribute to the establishment of the non-ETP TALL malignant clone remains to be investigated. Similarly, understanding how the other identified mutations alter the epigenetic landscape of a cell and contribute to transformation remains to be determined. This will require not only elucidating the effect of each mutation on the function of the encoded protein, but also determining how the mutant protein affects the epigenetic regulatory complexes in which it functions. This would require future investigation of how the altered function is influenced by the baseline epigenetic state of the target cell of transformation, and how this altered function complements other somatic mutations that are required for the development of overt cancer. The database developed by our work will help to focus further studies on the cell lineages that correspond to the tumour types in which specific mutations are detected. Patients and samples The use of human tissues for sequencing was approved by the institutional review boards of St Jude Children’s Research Hospital, Memorial Sloan-Kettering Cancer Center and Washington University in St Louis (St Jude IRB# FWA00004775, Protocol# XPD09-018). Written informed consent and/or assent were obtained from patients and/or legal guardians at the time of the surgical resection or bone marrow biopsy. Matched normal samples were obtained either from peripheral blood, bone marrow or adjacent normal tissue. All leukaemia samples have ≥70% blasts. The tumour content for the four subtypes of brain tumours, HGG, LGG, MB and EPD, exceeds 50, 67, 90 and 95%, respectively. The tumour purity for solid tumours ranges from 48 to 96%. Identification of genes involved in chromatin modification We searched multiple data sources to identify the proteins that: (1) bind a histone peptide, (2) modify nascent histone amino acids, (3) are part of established complexes involved in histone modification, (4) reorganize nucleosomes or (5) modify or bind modified genomic DNA. A core set of proteins was identified that is known to directly modify histones or DNA [13] , [27] , [28] , bind directly to modified or nascent histones [29] , [30] or alter chromatin state [31] . To expand our list to include additional homologues, we searched UniProt database [32] for the known histone reader domains (Bromo, Tandem Bromo, Chromo, PHD, Tandem PHD, Tudor, Tandem, PWWP, MBT, WD40, ADD, Ankyrin Repeats, ZF-CW and 14-3-3) [29] and catalytic modification domains (such as SET and Jumonji) [33] . The list was further expanded to include proteins within known complexes and potential complexes [15] , [16] , [17] , [18] , [19] , [20] , [21] , [22] , [31] . Potential epigenetic protein complexes were identified by using the core set of genes to search the STRING database (species=9,606 and required score >900) for interaction partners [34] . The large numbers of proteins identified were culled down by manually verifying that the interaction to a search protein was functionally relevant to histone, DNA modification or chromatin remodelling. All proteins were assigned a functional class (writers, erasers, reader, remodel chromatin, modify DNA, histone family, binding histone eraser and binding histone writer). In the case where proteins can be grouped in multiple classes, each protein was only assigned to the highest functional class available. Sequencing and experimental verification WGS ( n =434) and WES ( n =244), and analysis are described in detail elsewhere [6] , [7] . For 426 cases analysed by CC, libraries used for the enrichment were constructed from repli-G WGA DNA (Qiagen) with TruSeq DNA sample prep kits (Illumina), following manufacturer’s recommendations. Probe set for capturing all coding exons of the 633 chromatin-modifying genes was designed using Design Studio (Illumina). The resulting probe set was then synthesized and provided as part of a TruSeq Custom Enrichment kit (Illumina). Library hybridization and enrichment of the targeted regions was conducted using the manufacturer’s instructions. The enriched libraries were then sequenced on a HiSeq 2000 (Illumina) using V3 Chemistry (PE100 protocol), with 24 samples pooled per lane. Sequence data were analysed using the same methods as those for WGS and WES. For cases that were not subjected to WGS or WES, their TP53 mutation status was analysed by Sanger sequencing of coding exons using ABI3730 (Applied Biosystems). The majority of the putative variants were validated by NGS amplicon sequencing using the Nextera XT library prep kit (Illumina) and sequenced on the MiSeq (Illumina). Following an effective validation protocol [35] , the MiSeq paired-end 150-cycle protocol was performed with variants called by MiSeq reporter—a subset of the putative variants was validated by amplicon Sanger Sequencing using an ABI3730 and the BigDye 3.1 cycle sequencing kit (Applied Biosystems). Amplicons used for validation were generated from WGA DNA prepared independently of the material used for the custom enrichment, with oligos designed by software based on Primer3 (ref. 36 ). The PCR was performed with 20 ng of WGA DNA input using the AmpliTaq Gold 360 Master Mix (Life Technologies) as per the manufacturer’s instructions. Samples with existing WGS or WES data corroborating the SNVs or indels observed in the targeted enrichment data were considered to be validated. Functional and statistical significance of top 15 genes Loss-of-function mutations include indels or SNVs that result in frame shift, nonsense or affect splice sites. Functional significance of a missense mutation is determined for USP7 by majority rule (≥50% predict deleterious) using Polyphen [37] (probably_deleterious and greater), Sift [38] (deleterious) and Mutation Assessor [39] (medium assignment or greater). Known activating mutations were annotated based on literature search. Mutational significance was calculated for recurrently mutated genes. The background mutation rate (BMR) for WGS samples were estimated on the basis of mutations in non-coding, non-repetitive regions (that is, Tier3 data) and the disease-specific median BMR estimate was used for the BMR of WES and CC samples from the same disease type. The probability of a gene mutated in a specific sample under the null hypothesis of random background mutation was estimated from the amino-acid length and the BMR of the sample. The probability of observing a gene mutated in at least n samples under the null hypothesis of random background mutation was estimated using a one tail Poisson binomial distribution. Analysis of novel mutations in leukaemia To determine whether the mutations identified in leukaemia are novel, we first searched PubMed for all genes with recurrent SNVs with and without the term ‘cancer’. These genes were also used to mine the COSMIC data set v63 (downloaded 18 February 2013). To further classify novel genes within leukaemia, a similar PubMed search was performed with the search term ‘leukaemia’. This was accompanied by data mining of COSMIC to identify genes with mutations associated with the term ‘haematopoietic_and_lymphoid_tissue’. The associated publications were reviewed to determine whether the mutations in published literature were identified in paediatric or adult patients. Structural modelling and epigenetic regulator network The structure of the catalytic domain of USP7 ( Fig. 3b ) bound to ubiquitin aldehyde (PDB: 1NBF) was obtained from the PDB [26] , [40] . Mutations and graphics were generated using Pymol [41] . The network graph was generated in Cytoscape [42] . USP7 mutagenesis and transfection To demonstrate loss-of-function, two missense mutations identified in TALL (C300R and D305G) were introduced by site-direct mutagenesis (Agilent, Santa Clara, CA) on a wild-type USP7 cDNA construct (plasmid pCl-neo-Flag-HAUSP was deposited by Dr Bert Vogelstein at addgene). The following primers were used 5′-CATGATGTTCAGGAGCTTCGTCGAGTGTTGCTCGA-3′ for C300R-F and 5′-TCGAGCAACACTCGACGAAGCTCCTGAACATCATG-3′ for C300R-R, and 5′-GCTTTGTCGAGTGTTGCTCGGTAATGTGGAAAATAAGATGA-3′ for D305G-F and 5′-TCATCTTATTTTCCACATTACCGAGCAACACTCGACAAAGC-3′ for D305G-R. All constructs were sequenced for verification ( Supplementary Fig. 8 ). In all, 3 × 10 5 293T cells (ATCC, catalogue # CRL-11268) per well of a six-well plate were cultured in DMEM (Lonza, Walkersville, MD) with 10% of FBS (Sigma, Atlanta, GA). Two microgram of plasmid DNA was transfected into cells with X-tremeGENE HP DNA transfection reagent (Roche, Indianapolis, IN). Western blot Total protein of 293T cells was extracted at 72 h post transfection. Protein levels of USP7, total H2B and H2B ubiquityl Lys120 were detected by western blot with indicated antibodies. Human HAUSP (USP7) (catalogue # PA5-17179) and GAPDH (catalogue # MA5-15738) antibodies were purchased from Thermo Scientific (Rockford, IL), human H2B (catalogue # 39126) and H2BK120ub1 (catalogue # 39624) antibodies were purchased from Active Motif (Carlsbad, CA). Secondary goat anti-rabbit (catalogue # ab97051) or anti-mouse (catalogue # ab97265) antibodies were purchased from Abcam (Cambridge, MA). Briefly, the blots were incubated in the 1:1,000 diluted primary antibodies overnight at 4 °C and followed by incubating in 1:5,000 diluted secondary antibodies. The protein bands were detected by SuperSignal West Femto Maximum Sensitivity Substrate (catalogue # 34096) purchased from Thermo Scientific (Rockford, IL). Accession codes: Sequence data for the paediatric cancer samples in this study have been deposited in the EBI-EMBL EGA under the accession code EGAS00001000449. How to cite this article: Huether, R. et al. The landscape of somatic mutations in epigenetic regulators across 1,000 paediatric cancer genomes. Nat. Commun. 5:3630 doi: 10.1038/ncomms4630 (2014).